Gate sequence for continuous variable one-way quantum computation Measurement-based one-way quantum computation using cluster states as resources provides an efficient model to perform computation and information processing of quantum codes. Arbitrary Gaussian quantum computation can be implemented sufficiently by long single-mode and two-mode gate sequences. However, continuous variable gate sequences have not been realized so far due to an absence of cluster states larger than four submodes. Here we present the first continuous variable gate sequence consisting of a single-mode squeezing gate and a two-mode controlled-phase gate based on a six-mode cluster state. The quantum property of this gate sequence is confirmed by the fidelities and the quantum entanglement of two output modes, which depend on both the squeezing and controlled-phase gates. The experiment demonstrates the feasibility of implementing Gaussian quantum computation by means of accessible gate sequences. Measurement-based one-way quantum computation (QC) performs computation by measurement and classical feedforward on a multipartite cluster entangled state [1] . One-way QC was first demonstrated using four-photon cluster states [2] , [3] . Besides photonic systems [2] , [3] , [4] , [5] , [6] , other QC systems with discrete quantum variables, such as ionic [7] , [8] , [9] , [10] , superconducting [11] , [12] , [13] , [14] , [15] and solid state [16] , [17] , [18] systems, have been investigated. In parallel, the theoretical and experimental explorations on one-way continuous variable (CV) QC have also been developed [19] , [20] , [21] , [22] , [23] , [24] , [25] , [26] , [27] , [28] , [29] , [30] . In contrast to the probabilistic generation of photonic qubits in most cases, CV cluster states are produced in an unconditional fashion and thus the one-way QC with CV cluster states can be implemented deterministically [27] , [28] , [29] , [30] , [31] , [32] , [33] , [34] . Although individual single-mode and two-mode logical gates towards implementing multimode Gaussian transformation in a one-way CVQC fashion have been experimentally demonstrated by using four-mode cluster entangled states of light [27] , [28] , [29] , [30] , CV gate sequences consisting of different single logical elements, which are necessary for realizing practical QC, have not been reported up to now. It is now important to investigate the gate sequences for QC as sufficiently large cluster states have recently been prepared, including eight-photon [35] , [36] , eight-quantum mode [37] , [38] and up to 10,000-quantum mode [39] optical cluster states. Here, we design and experimentally accomplish a CV gate sequence, in which a single-mode squeezing gate and a two-mode controlled-phase (CZ) gate are cascaded. A vacuum optical input signal is first squeezed by the squeezing gate and successively the squeezed output enters the CZ gate as one of its two inputs. A vacuum state or a squeezed state of light produced by an off-line nondegenerate optical parametric amplifier (NOPA) is used for the other CZ gate input. The experimental result shows that after two independent input states are transformed by the gate sequence, the two output states produced are entangled and their fidelities are better than that obtained by using coherent states as resources. Our experiments also prove that the entanglement degree and the fidelity depend simultaneously on two cascaded logical gates, which manifests the sequence feature of the presented system. Apart from the gate sequences only involving multimode Gaussian transformation, a non-Gaussian operation is required at least [19] for demonstrating universal one-way CVQC. Many theoretical protocols and schemes on the universal CVQC have been proposed [19] , [20] . Preparation of six-mode CV cluster states CV cluster states are defined as [21] , [22] In the limit of infinite squeezing, the N -mode cluster states are a simultaneous zero eigenstate of the N linear combinations in equation (1). Here the amplitude ( ) and phase ( ) quadratures of an optical mode are defined as and . The modes a ∈ G denote the vertices of the graph G , while the modes b ∈ N a are the nearest neighbours of mode . One time measurement on the cluster state cannot destroy the entanglement totally, which means that cluster states have strong properties of entanglement persistence. A general way to build CV cluster states is to implement an appropriate unitary transformation ( U ) on a series of input -squeezed states, , where r is the squeezing parameter, and represent the quadratures of a vacuum state, which has a noise variance . According to a general linear optics transformation , the output modes can be obtained [22] . The transformation matrix U can be decomposed into a network of beam-splitters, which corresponds to the experimental system for generating the required CV cluster state. We designed the beam-splitter network for producing CV six-mode linear cluster states with three NOPAs, as shown in Fig. 1 . A NOPA can simultaneously generate a -squeezed state and a -squeezed state [40] . The three -squeezed states and three -squeezed states prepared by the three NOPAs, are denoted by , ,( m =1, 3, 5) for -squeezed states, and , , ( n =2, 4, 6) for -squeezed states, respectively. Here we have assumed that all squeezed states produced by the three NOPAs have identical squeezing degree due to the equality of their configuration (see Methods). 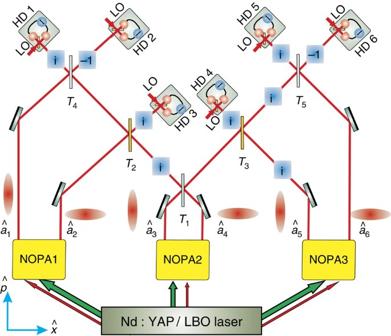Figure 1: Schematic of six-mode CV cluster state generation system. T: transmission efficient of beam splitter. Boxes including aniare Fourier transforms (90° rotations in phase space), and −1 is a 180° rotation. LO, local oscillation beam; HD, homodyne detector. We deduce the transformation matrix for generating CV six-mode linear cluster state using three -squeezed states and three -squeezed states as input states, which is given by [22] Figure 1: Schematic of six-mode CV cluster state generation system. T : transmission efficient of beam splitter. Boxes including an i are Fourier transforms (90° rotations in phase space), and −1 is a 180° rotation. LO, local oscillation beam; HD, homodyne detector. Full size image The matrix can be decomposed into , where F k denotes the Fourier transformation of mode k , which corresponds to a 90° rotation in the phase space; stands for the linearly optical transformation on the j th beam-splitter with the transmission of T j ( j =1,…,5), where , , , and are elements of beam-splitter matrix. I k (−1)= e i π corresponds to a 180° rotation of mode k in phase space. When the transmissions of the five beam-splitters are chosen as T 1 =9/13, T 2 = T 3 =1/3, T 4 = T 5 =1/2, the six output optical modes construct a six-mode CV linear cluster state. The corresponding excess noise terms for each mode of the CV six-mode linear cluster state are respectively denoted by Obviously, in the ideal case with infinite squeezing ( r →∞), these excess noises will vanish and the better the squeezing, the smaller the noise term will be. 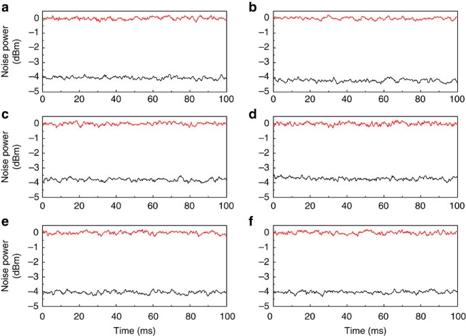Figure 2: Measured correlation noises of six-mode CV cluster state. Panelsa–fare noise powers of,,,,and, respectively. The red and black lines in all plots are shot-noise level and correlation variances, respectively. Measurement frequency is 2 MHz, the spectrum analyser resolution bandwidth is 30 kHz and the video bandwidth is 100 Hz. Figure 2 shows the experimental results of the six-mode CV cluster state. Red and black lines correspond to shot-noise level (SNL) and quantum correlation noise, respectively. The measured noises are =−4.04±0.09 dB, =−4.22±0.10 dB, =−3.80±0.10 dB, =−3.72±0.09 dB, =−4.05±0.10 dB, and =−4.03±0.09 dB, respectively. Figure 2: Measured correlation noises of six-mode CV cluster state. Panels a–f are noise powers of , , , , and , respectively. The red and black lines in all plots are shot-noise level and correlation variances, respectively. Measurement frequency is 2 MHz, the spectrum analyser resolution bandwidth is 30 kHz and the video bandwidth is 100 Hz. Full size image According to the inseparability criteria for CV multipartite entangled states proposed by van Loock and Furusawa [41] , we deduced the inseparability criteria for CV six-partite linear cluster state, which are Substituting the measured quantum noise ( Fig. 2 ) into equations (4)–(8), we can calculate the combinations of the correlation variances, which are 0.48, 0.59, 0.63, 0.62 and 0.50, respectively. As all these values are smaller than the boundary of 1, the prepared six quantum modes satisfy the inseparability criteria and form a six-mode cluster entangled state. Configuration of the gate sequence As shown in Fig. 3a , we demonstrate the gate sequence of a squeezing gate and a CZ gate using a six-mode cluster state as ancillary state. First, we perform the squeezing gate on input mode α (target mode) to produce a phase-squeezed state. Then a CZ gate is performed on the output mode from the squeezing gate and the other input mode β (control mode) coming from outside of the sequence. 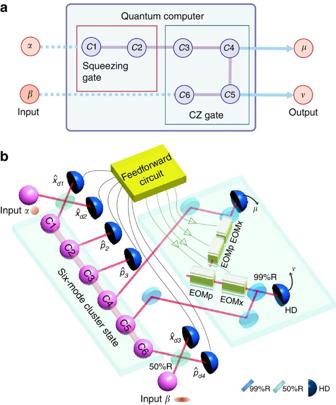Figure 3: Schematic of the gate sequence. (a) The graph representation. The input stateαis coupled to a six-mode CV cluster stateC1-C2-C3-C4-C5-C6. Squeezing operation is performed on input modeα, then CZ gate is performed on the input stateβand output of the squeezing operation. (b) Schematic of the experimental setup. The input statesαandβare coupled to a six-mode CV cluster state via 50% beam-splitter (50%R). Measurement results from HD systems are fed forward to modesC4 andC5. The output modesμandνare measured by two HD systems. EOMx and EOMp: amplitude and phase EOM. 99%R, a mirror with 99% reflection coefficient. Figure 3: Schematic of the gate sequence. ( a ) The graph representation. The input state α is coupled to a six-mode CV cluster state C 1- C 2- C 3- C 4- C 5- C 6. Squeezing operation is performed on input mode α , then CZ gate is performed on the input state β and output of the squeezing operation. ( b ) Schematic of the experimental setup. The input states α and β are coupled to a six-mode CV cluster state via 50% beam-splitter (50%R). Measurement results from HD systems are fed forward to modes C 4 and C 5. The output modes μ and ν are measured by two HD systems. EOMx and EOMp: amplitude and phase EOM. 99%R, a mirror with 99% reflection coefficient. Full size image The single-mode squeezing gate is expressed by . The input–output relation of the single-mode squeezing gate is , where and represents the squeezing operation on phase quadrature. The CV CZ gate corresponds to the unitary operator with the input–output relation, where , and I is a 2 × 2 identity matrix. The transformation matrix of the gate sequence is given by The input–output relation of the gate sequence is expressed by in the ideal case. However, in any practical cases, the excess noise coming from imperfect entanglement of the CV cluster state will inevitably affect the performances of the logical gates, thus a noise term should be added, that is where represents all excess noises of the gate sequence. The schematic of experimental setup is shown in Fig. 3b . A six-mode cluster state involving six submodes C 1, C 2, C 3, C 4, C 5 and C 6 with the squeezing about −4.0 dB on average is used as the resource (ancillary) state. The input states α and β are coupled to submodes C 1 and C 6 by two 50% beam-splitters, respectively. The measurement results of the output modes from the two 50% beam-splitters as well as the submodes C 2 and C 3 are feedforward to submodes C 4 and C 5 through classical feedforward circuits. In the operation of gate sequence, the measured observables are , , , , and . The measurement angle θ 1 and θ 2 in the homodyne detection for and determine the squeezing operation according to the transformation matrix if we choose θ 2 =− θ 1 . S corresponds to a single-mode amplitude and phase squeezing gate when cot θ 2 = and , respectively. The measurement angles ( θ 1 , θ 2 ) for 0 dB, −3 dB, −6 dB, −9 dB and −12 dB squeezing are (−45.00°, 45.00°), (−35.30°, 35.30°), (−26.62°, 26.62°), (−19.54°, 19.54°), and (−14.10°, 14.10°), respectively. These measurement results are feedforwarded to the amplitude and phase quadratures of modes C 4 and C 5 via electro-optical modulators (EOM), respectively. The corresponding feedforward operation is expressed by , where and are the amplitude and phase displacement operators, respectively, , , , and . The output modes are detected by two homodyne detection systems. The quadrature components of the output modes for the gate sequence are given by where is the feedforward gain factor. From equations (14) and (15) we obtain After a vacuum signal ( α ) passes through the squeezing gate, its phase ( ) and amplitude ( ) are squeezed ( ) and anti-squeezed ( ), respectively. Then, the squeezed signal passes through the CZ gate, as the usual result of CZ gate [30] , the anti-squeezed amplitude signal is transformed into the phase quadrature ( ) of the resultant output mode ν and its amplitude quadrature ( ) keeps unchanging in the ideal case without excess noises ( =0). Experimental results As a CZ gate is a two-mode entangling gate, its quantum character can be verified by the sufficient condition of inseparability for a two-mode state [42] , that is where g is the optimal gain factor, which makes the left side of the inequality minimum. By calculating the minimal value of equation (18), the optimal gain is obtained where r β is the squeezing parameter of the input mode β . 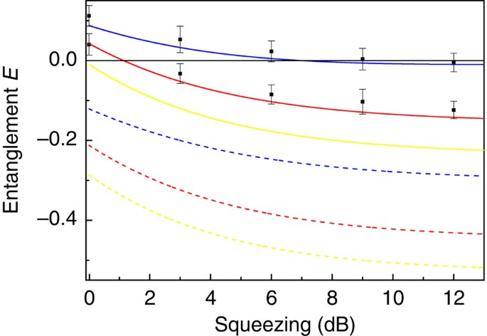Figure 4: Dependence of entanglement on squeezing of the squeezing gate. The dependence of the entanglement between the gate sequence output modes on the squeezing of the squeezing gate is plotted here. The blue, red and yellow lines correspond to the input mode β being a vacuum state, −4 dB and −12 dB phase-squeezed state, respectively. The solid and dashed lines correspond to −4 dB and −6 dB squeezing of the six-mode cluster state, respectively. The black dots represent the experimental data. Error bars represent±one s.d. and are obtained based on the statistics of the measured noise variances. Figure 4 shows the dependence of entanglement degree between the two output states of the gate sequence on squeezing degree of the squeezing gate with an input vacuum mode α for three different β states (blue: vacuum state, red: −4 dB phase-squeezed state, yellow: −12 dB phase-squeezed state). The entanglement degree is quantified by . When E <0, the entanglement exists and the smaller the E , the stronger the entanglement. The solid and dashed lines correspond to −4 and −6 dB squeezing of the six-mode cluster state, respectively. All traces are plotted according to the real loss in our experimental system (see Methods). We can see that the entanglement degree between the output states ( μ and ν ) not only depends on the operation of CZ gate, but also is controlled by the squeezing operation of the squeezing gate. For a given β state, when the squeezing of the squeezing gate increases, the entanglement degree of the output states increases. On the other hand, the operation of the CZ gate also depends on the features of the β state. The phase squeezing of the β state will improve the entanglement degree of the output modes. Of course, the largest influence to the capacity of the gate sequence comes from the quality of the resource state. When the squeezing of the six-mode cluster state increases from −4 dB (solid lines) to −6 dB (dashed lines), the entanglement degree of the output states will be significantly improved. As −4 dB cluster squeezing is available in our experiment, the obtained maximal entanglement degree is only −0.005 for the case of using two vacuum states to be α and β (solid blue line). If β is a phase-squeezed state (red and yellow lines), the entanglement will increase for the same squeezing degree of the squeezing gate and an identical resource state. The experimentally measured data points obtained under different measurement angles of the squeezing gate are marked by little black dots with error bars, which shows that the experimental results are in reasonable agreement with the theoretical expectation. The experimentally measured entanglement degrees, fidelities and corresponding optimal gain factors are listed in Table 1 . The entanglement degree of the output modes depends on both operations of two cascaded gates, which clearly shows that the final results are decided by the gate sequence. Figure 4: Dependence of entanglement on squeezing of the squeezing gate. The dependence of the entanglement between the gate sequence output modes on the squeezing of the squeezing gate is plotted here. The blue, red and yellow lines correspond to the input mode β being a vacuum state, −4 dB and −12 dB phase-squeezed state, respectively. The solid and dashed lines correspond to −4 dB and −6 dB squeezing of the six-mode cluster state, respectively. The black dots represent the experimental data. Error bars represent±one s.d. and are obtained based on the statistics of the measured noise variances. Full size image Table 1 Entanglement and fidelity at experimentally measured data point s . 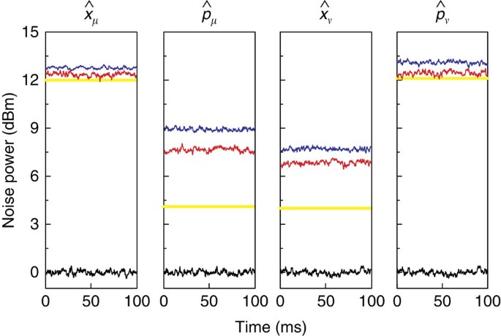Figure 5: Experimentally measured noise powers. The measured noise powers of the output modes with a vacuum and a phase-squeezed state as inputs are plotted here. Black lines are SNL, blue and red lines are output noise power without and with cluster state as ancillary state, yellow lines are ideal output noise power. Squeezing degree of the squeezing gate is −12 dB. Measurement frequency is 2 MHz, the spectrum analyser resolution bandwidth is 30 kHz and the video bandwidth is 100 Hz. Full size table Figure 5 shows the measured noise variances of the quadratures ( , , , and ) of the output modes ( μ and ν ) with a vacuum mode α and a phase-squeezed state β with squeezing of −4 dB as two inputs of the gate sequence, where −12 dB squeezing is implemented on input α . In the ideal case with the cluster state of infinite squeezing (yellow lines), the noise powers of and are 12 and 4 dB above the SNL (black lines), which correspond to the anti-squeezing noises resulting from the squeezing gate (12 dB) and the input phase-squeezed state (4 dB), respectively. The noise powers of and are 4.1 and 12.1 dB above the SNL due to the effect of CZ gate (see equation (17)). The blue and red lines stand for the output noises without and with the cluster state as ancillary state, respectively. The blue lines are obtained by using a coherent light of identical intensity to replace each of cluster submodes. In this case, the measured values of , , , and are 12.75±0.07, 9.05±0.09, 7.76±0.08 and 13.07±0.09 dB above the SNL, respectively. The noise variances of , , , and measured with the existence of the cluster state (red lines) are 12.34±0.11, 7.60±0.13, 6.84±0.12 and 12.55±0.13 dB above the SNL, respectively, all of which are lower than the corresponding values without using the cluster resource. Figure 5: Experimentally measured noise powers. The measured noise powers of the output modes with a vacuum and a phase-squeezed state as inputs are plotted here. Black lines are SNL, blue and red lines are output noise power without and with cluster state as ancillary state, yellow lines are ideal output noise power. Squeezing degree of the squeezing gate is −12 dB. Measurement frequency is 2 MHz, the spectrum analyser resolution bandwidth is 30 kHz and the video bandwidth is 100 Hz. Full size image To further verify the general input–output relation of the gate sequence, we employ a coherent state with a 15 dB modulation signal as input state ( Fig. 6a–d ). 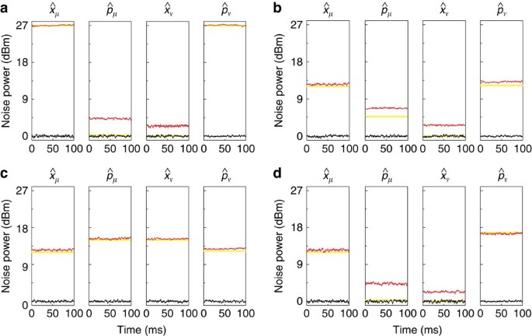Figure 6: Experimentally measured noise powers of the output modes with coherent inputs. (a–d):,,and-coherent state as input, respectively. Black lines are SNL, red lines are output noise power with cluster state as ancillary state, yellow lines are ideal output noise power. Squeezing degree of the squeezing gate is −12 dB. Measurement frequency is 2 MHz. The spectrum analyser resolution bandwidth is 30 kHz and the video bandwidth is 100 Hz. Figure 6a shows the noise powers of quadratures of the output modes μ and ν when input modes α and β are a coherent state with nonzero amplitude of 15 dB ( -coherent) and a vacuum state, respectively. The measured noise variance of (red line) is 27.01±0.13 dB above SNL (black lines). That is because 12 dB anti-squeezing noise resulting from the squeezing gate is added on the 15 dB input amplitude of . In the ideal case (yellow lines), the noise variance of is a little higher than SNL as is added on the squeezed noise of −12 dB, and the noise variance of is at the level of SNL. The measured noise powers of and is about 4.43±0.16 and 2.68±0.18 dB above the SNL because of the effect of excess noises coming from the imperfect entanglement of the cluster state. The measured noise variance of is 27.02±0.11 dB above the SNL because the amplitude on is added to , which satisfies the input–output relation of the CZ logic gate in equation (17). Figure 6b shows the noise powers of output modes when a coherent state with a modulation signal of 15 dB on ( -coherent) and a vacuum state are used for the input states α and β , respectively. The measured noise power (red lines) of is 12.34±0.17 dB above the corresponding SNL (black line) because of the effect of anti-squeezing noise resulting from the squeezing gate. The noise powers of and (red lines) are 6.72±0.12 dB and 2.68±0.12 dB above the corresponding SNL, respectively. The noise power of is 12.68±0.14 dB above the SNL because the noise of is added on (see equation (17)). Figure 6c,d are the noise powers of output modes when the input is the coherent state with the modulation signal of 15 dB on and ( -coherent and -coherent), respectively. It is obvious that the measured noise powers of output modes satisfy the input–output relation of the gate sequence in equation (17). Figure 6: Experimentally measured noise powers of the output modes with coherent inputs. ( a – d ): , , and -coherent state as input, respectively. Black lines are SNL, red lines are output noise power with cluster state as ancillary state, yellow lines are ideal output noise power. Squeezing degree of the squeezing gate is −12 dB. Measurement frequency is 2 MHz. The spectrum analyser resolution bandwidth is 30 kHz and the video bandwidth is 100 Hz. 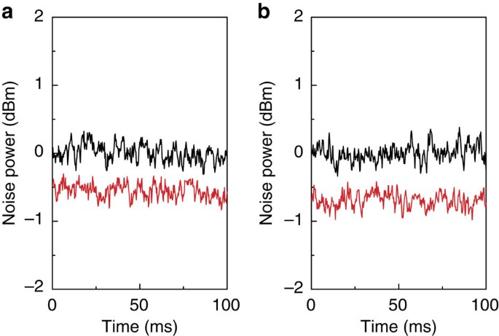Figure 7: Measured quantum correlation variances. This figure show the measured quantum correlation variances of the output modes of the gate sequence with a vacuum state and a phase-squeezed state as inputs.aandbare noise power ofand, respectively. Black and red lines are SNL and quantum correlation noise, respectively. Squeezing degree of the squeezing gate is −12 dB. Measurement frequency is 2 MHz, the spectrum analyser resolution bandwidth is 30 kHz and the video bandwidth is 100 Hz. Full size image Figure 7 shows the measured correlation noise variances of the output modes with a vacuum mode ( α ) and a −4 dB phase-squeezed mode ( β ) as the inputs of the sequence, where −12 dB squeezing is implemented on input α . The measured noise variance (red lines) of (a) and (b) are 0.53±0.11 and 0.65±0.11 dB below the corresponding SNL (black lines), respectively. The entanglement is quantified by Figure 7: Measured quantum correlation variances. This figure show the measured quantum correlation variances of the output modes of the gate sequence with a vacuum state and a phase-squeezed state as inputs. a and b are noise power of and , respectively. Black and red lines are SNL and quantum correlation noise, respectively. Squeezing degree of the squeezing gate is −12 dB. Measurement frequency is 2 MHz, the spectrum analyser resolution bandwidth is 30 kHz and the video bandwidth is 100 Hz. Full size image For our experimental system, the calculated optimal gain factor is g =0.98. The total correlation variances in the left side of equation (18) are smaller than g and thus satisfy the inseparability criteria, which confirms the quantum entanglement between the two output modes ( μ and ν ) from the gate sequence. We also use fidelity , which denotes the overlap between the experimentally obtained output state and the ideal output sate , to quantify the performance of the gate sequence. The fidelity for two Gaussian states and with covariance matrices A j and mean amplitudes α j ≡( α jx , α jp ) ( j =1,2) is expressed by [43] , [44] where Δ=det( A 1 + A 2 ), σ =(det A 1 −1)(det A 2 −1), = α 2 − α 1 , A 1 and A 2 for the ideal ( ) and experimental ( ) output states, respectively. The covariance matrices A j ( j =1, 2) for target mode are given by The coefficient ‘4’ comes from the normalization of SNL. As the noise of a vacuum state is defined as 1/4, while in the fidelity formula the vacuum noise is normalized to ‘1’, a coefficient ‘4’ appears in the expressions of covariance matrices. Similarly, we can write out the covariance matrices for the control mode In case of infinite squeezing, both fidelities for the target and control states, F μ and F ν , equal to 1, which can be calculated from equation (17) with r → ∞. 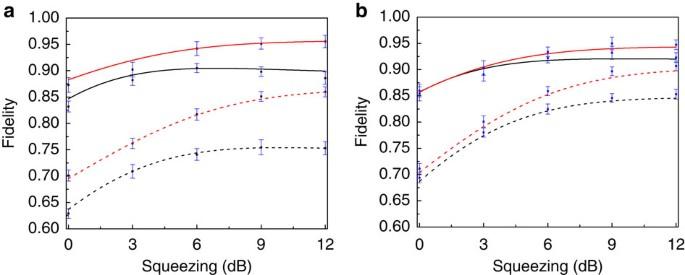Figure 8: Dependence of fidelity on squeezing of the squeezing gate. aandbare the fidelity for the input modeβas a vacuum state and a −4 dB phase-squeezed state, respectively. The solid and dashed lines correspond to fidelity with and without cluster resource, respectively. Black and red lines present the fidelity of output modesμandν, respectively. Error bars represent±one s.d. and are obtained based on the statistics of the measured noise variances. Figure 8 gives the fidelities of the output modes μ and ν, as the function of squeezing degree of the squeezing gate based on the experimental data for two different input β states ( Fig. 8a is a vacuum state; Fig. 8b is a −4 dB phase-squeezed state). In Fig. 8 , black and red lines correspond to fidelity of output modes μ and ν, respectively. Dashed lines are obtained at the case without the use of the cluster resource (using the coherent states in the same intensity to substitute the cluster states in Fig. 3 ) and solid lines are completed under the case using the cluster resource state. Obviously, when the cluster state is applied, the fidelity of the output states is higher than that obtained at the case using the coherent state, which is usually called the classical limit in quantum optics. The experimentally measured data (see Table 1 ) are marked in Fig. 8a,b , and are in reasonable agreement with the theoretical calculation. Figure 8: Dependence of fidelity on squeezing of the squeezing gate. a and b are the fidelity for the input mode β as a vacuum state and a −4 dB phase-squeezed state, respectively. The solid and dashed lines correspond to fidelity with and without cluster resource, respectively. Black and red lines present the fidelity of output modes μ and ν , respectively. Error bars represent±one s.d. and are obtained based on the statistics of the measured noise variances. Full size image We demonstrated a gate sequence in one-way QC fashion by applying a six-mode CV cluster state as quantum resource. The quantum feature of the gate sequence is verified quantitatively by both the inseparability criterion of two-mode entanglement and the fidelities of output states. The entanglement degree of two output modes depends on two cascaded gates, simultaneously, which exhibits the sequence character of the system. Although in our experiment only two gates are linked together, the scheme can be easily extended to construct any large QC gate sequence with a number of gates. Today, quantum computers have become a physical reality and are continuing to be developed. One-way QC based on quantum teleportation [23] , [24] is able to implement secure information processing and accomplish the unbreakable quantum coding [45] , [46] . On the other hand, the large cluster states can be prepared only by linearly optical systems if appropriate squeezed states are available. Thus, one-way quantum computers consisting of this type of gate sequences can be operated in a reverse blind CVQC model to realize the secure QC network ( Fig. 9 ), in which only a server owns the ability of preparing quantum states (such as squeezed states) and all remote clients ask the server to send them necessary squeezed states through a quantum channel [47] . Then, clients produce the cluster states using linearly optical transformation and perform arbitrary CV one-way Gaussian QC by means of classical measurements and feedforwards on the prepared cluster state at their stations. In this way, the server and any eavesdroppers never know what clients want to do, thus the security of the blind QC is guaranteed by no-signaling principle [48] . The presented gate sequence for one-way Gaussian CVQC is an essential experimental exploration towards developing universal QC and practical quantum networks. 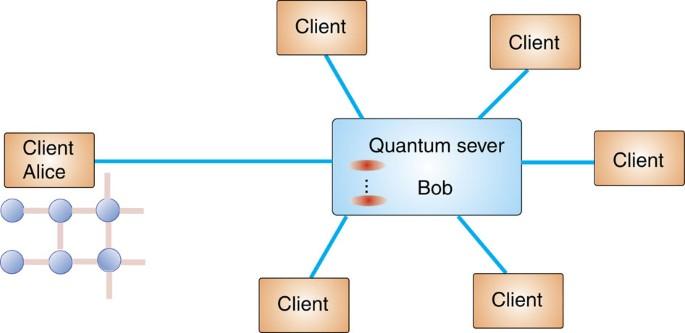Figure 9: Schematic of reverse blind CVQC. The quantum server prepares squeezed states and sends them to any clients in demand. Client prepares CV cluster state with linear optics and then implements quantum computation via measurements and feedforwards on the prepared cluster state. Figure 9: Schematic of reverse blind CVQC. The quantum server prepares squeezed states and sends them to any clients in demand. Client prepares CV cluster state with linear optics and then implements quantum computation via measurements and feedforwards on the prepared cluster state. Full size image Experimental details The three -squeezed and three -squeezed states are produced by three NOPAs. These NOPAs are pumped by a common laser source, which is a continuous wave intracavity frequency-doubled and frequency-stabilized Nd:YAP/LBO(Nd-doped YAlO 3 perorskite/lithium triborate) [49] . The output fundamental wave at 1,080 nm wavelength from the laser is used for the injected signals of NOPAs and the local oscillators of the homodyne detectors. The output second harmonic wave at 540 nm wavelength serves as the pump field of all NOPAs, in which a pair of signal and idler modes with the identical frequency at 1,080 nm and the orthogonal polarizations are generated through an intracavity frequency-down-conversion process [50] . Each of NOPAs consists of an α-cut type-II KTP crystal and a concave mirror [50] . The front face of the KTP was coated to be used for the input coupler and the concave mirror serves as the output coupler of the squeezed states, which is mounted on a piezo-electric transducer (PZT) for locking actively the cavity length of NOPA on resonance with the injected signal at 1,080 nm. The transmissions of the input coupler at 540 nm and 1,080 nm are 99.8% and 0.04%, respectively. The transmissions of the output coupler at 540 nm and 1,080 nm are 0.5% and 5.2%, respectively. The finesses of the NOPA for 540 nm and 1,080 nm are 3 and 117, respectively. In our experiment, all NOPAs are operated at the parametric deamplification situation, that is, the phase difference between the pump field and the injected signal is (2 n +1)π ( n is an integer). Under this condition, the coupled modes at +45° and −45° polarization directions are the quadrature amplitude and the quadrature phase-squeezed states, respectively [31] , [40] . Three NOPAs are locked individually by means of Pound-Drever-Hall method with a phase modulation of 56 MHz on 1,080 nm laser beam [51] . In the experiment, the relative phase (2 n +1)π locking is completed with a lock-in amplifier, where a signal around 15 kHz is modulated on the pump light by the PZT mounted on a reflection mirror, which is placed in the optical path of the pump laser and then the error signal is fed back to the other PZT, which is mounted on a mirror placed in the optical path of the injected beam. In the beam-splitter network used to prepare six-mode cluster states, the relative phase between two incident beams on T 1 and T 4 is phase-locked to zero, and that on T 2 , T 3 and T 5 is phase-locked to π/2. The zero phase difference ( T 1 and T 4 ) between two interfered beams on a beam-splitter is locked by a lock-in amplifier. The π/2 phase difference ( T 2 , T 3 and T 5 ) is locked by DC locking technique, where the photocurrent signal of the interference fringe is fed back to the PZT mounted on a mirror, which is placed before the beam-splitter. In the homodyne detection system, zero phase difference for the measurement of quadrature amplitude is locked by Pound-Drever-Hall technique with a phase modulation of 10.9 MHz on local oscillator beam. The π/2 phase for the measurement of quadrature phase is locked with DC locking technique too. The transmission efficiency of an optical beam from NOPA to a homodyne detector is around 96%. The quantum efficiency of a photodiode (FD500W-1064, Fermionics) used in the homodyne detection system is 95%. The interference efficiency on a beam-splitter is about 99%. The phase fluctuation of the phase locking system is about 2–3°. How to cite this article: Su, X. et al . Gate sequence for continuous variable one-way quantum computation. Nat. Commun. 4:2828 doi: 10.1038/ncomms3828 (2013).